CCM-3/STRIPAK promotes seamless tube extension through endocytic recycling The mechanisms governing apical membrane assembly during biological tube development are poorly understood. Here, we show that extension of the C. elegans excretory canal requires cerebral cavernous malformation 3 (CCM-3), independent of the CCM1 orthologue KRI-1. Loss of ccm-3 causes canal truncations and aggregations of canaliculular vesicles, which form ectopic lumen (cysts). We show that CCM-3 localizes to the apical membrane, and in cooperation with GCK-1 and STRIPAK, promotes CDC-42 signalling, Golgi stability and endocytic recycling. We propose that endocytic recycling is mediated through the CDC-42-binding kinase MRCK-1, which interacts physically with CCM-3–STRIPAK. We further show canal membrane integrity to be dependent on the exocyst complex and the actin cytoskeleton. This work reveals novel in vivo roles of CCM-3·STRIPAK in regulating tube extension and membrane integrity through small GTPase signalling and vesicle dynamics, which may help explain the severity of CCM3 mutations in patients. Multicellular organisms contain myriad biological tubes that transport gases and fluids within organs and throughout the body. These tubes can develop through a variety of mechanisms, such as wrapping, cavitation and cell hollowing [1] , [2] . The mechanism of lumen formation, and regulation of tube diameter, is dependent on whether the tube is multicellular, autocellular or seamless. Seamless tubes are unicellular, do not have junctions and form by the process of cell hollowing [2] . Proper control of tube length and diameter is of fundamental importance during development, and defects can lead to pathologies, such as polycystic kidney disease and cerebral cavernous malformations (CCMs) [3] , [4] . Genetically tractable organisms (for example, the fruit fly Drosophila melanogaster and the nematode Caenorhabditis elegans ) have revealed conserved mechanisms by which biological tubes develop and how their integrity is maintained [1] , [5] , [6] . The excretory canal is a seamless unicellular tube that maintains osmotic balance and ion levels in C. elegans [6] , [7] . Created in the embryo, the excretory cell projects two arms dorsolaterally until they reach the hypodermis, where they bifurcate and extend bi-directionally along the anterior/posterior axis, forming two long canals ( Fig. 1a ). As seen in a cross-section ( Fig. 1b ), canals are comprised of a basal (outer) membrane, a cytoplasmic region containing canalicular vesicles (CVs), organelles (endoplasmic reticulum (ER), Golgi and mitochondria), and an apical (inner) membrane that envelops the lumen. During its post-embryonic extension phase, actin-based projections stimulate outgrowth of the canal tip causing the excretory canal to undergo marked morphological changes [6] . It is thought that lumen formation and extension of the apical (luminal) membrane is the driving force of tubulogenesis, but how membrane is added during this growth phase is presently not well understood. The canals of lumen defective mutants do not extend and show accumulation and hyperfusion of CVs in the cytoplasmic space, which reveals important links between these membrane sources and canal morphology [8] , [9] . 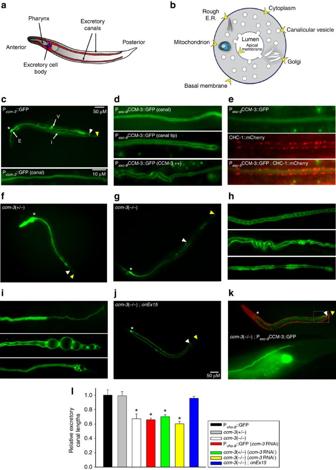Figure 1: Loss ofccm-3affects canal growth. (a)C. elegansexcretory canals connect below the posterior bulb of the pharynx, extending two arms in anterior and posterior directions that create a distinctive ‘H’ shape. (b) Cross-sectional view of the canal depicts a basal membrane and cytoplasmic space in which membranous channels (canalicular vesicles, CVs) aggregate and fuse to form the lumen. Mitochondria, Golgi and ER are distributed along the length of wild-type canals. (c) Theccm-3promoter fused to GFP shows robust expression in the intestine (I), vulva (V) and excretory canals (E). (d) A canal-specific translational reporter indicates CCM-3 presence in the cytoplasm, and a strong enrichment at the apical membrane. Overexpression of CCM-3 causes a misshapen canal with a widened lumen (bottom panel). (e) Apical enrichment is confirmed through a co-localization with CHC-1 (a basolateral marker). While no canal defects (canal marked with Pvha-8::GFP) are evident with loss of one copy ofccm-3(f), loss of both copies causes canal truncations (g,l) and lumen defects (including cyst formation) along the length of the canal (h), and at the distal tip (i). Expression of CCM-3 from its endogenous promoter fully rescues canal truncations inccm-3(−/−) (j,l), while expressing CCM-3 using the canal-specificexc-9promoter (indicated by the red signal of co-injection marker) rescued canals inccm-3(−/−) to wild-type length (region marked by an inset box) (k,l). In addition,ccm-3(RNAi)causes truncation in the canal like the homozygous mutation (l). Asterisks denote location of the excretory cell (at the anterior/head of the worm), white and yellow arrowheads denote canal and total worm length, respectively. All canals are oriented from anterior (left) to posterior (right).c(top),f,g,jandk(top) are at × 100 magnification;c(bottom),d,e,h,iandk(bottom) are at × 630 magnification. Scale bars are indicated for whole worm and high-magnification canal sections in the first appropriate panel, and are modified only in panels where the magnification is different. Graph shows average ±s.e.m.,n≥60, *P<0.05 versus control (Student’st-test). Figure 1: Loss of ccm-3 affects canal growth. ( a ) C. elegans excretory canals connect below the posterior bulb of the pharynx, extending two arms in anterior and posterior directions that create a distinctive ‘H’ shape. ( b ) Cross-sectional view of the canal depicts a basal membrane and cytoplasmic space in which membranous channels (canalicular vesicles, CVs) aggregate and fuse to form the lumen. Mitochondria, Golgi and ER are distributed along the length of wild-type canals. ( c ) The ccm-3 promoter fused to GFP shows robust expression in the intestine (I), vulva (V) and excretory canals (E). ( d ) A canal-specific translational reporter indicates CCM-3 presence in the cytoplasm, and a strong enrichment at the apical membrane. Overexpression of CCM-3 causes a misshapen canal with a widened lumen (bottom panel). ( e ) Apical enrichment is confirmed through a co-localization with CHC-1 (a basolateral marker). While no canal defects (canal marked with P vha-8 ::GFP) are evident with loss of one copy of ccm-3 ( f ), loss of both copies causes canal truncations ( g , l ) and lumen defects (including cyst formation) along the length of the canal ( h ), and at the distal tip ( i ). Expression of CCM-3 from its endogenous promoter fully rescues canal truncations in ccm-3(− /−) ( j , l ), while expressing CCM-3 using the canal-specific exc-9 promoter (indicated by the red signal of co-injection marker) rescued canals in ccm-3(− /−) to wild-type length (region marked by an inset box) ( k , l ). In addition, ccm-3(RNAi) causes truncation in the canal like the homozygous mutation ( l ). Asterisks denote location of the excretory cell (at the anterior/head of the worm), white and yellow arrowheads denote canal and total worm length, respectively. All canals are oriented from anterior (left) to posterior (right). c (top), f , g , j and k (top) are at × 100 magnification; c (bottom), d , e , h , i and k (bottom) are at × 630 magnification. Scale bars are indicated for whole worm and high-magnification canal sections in the first appropriate panel, and are modified only in panels where the magnification is different. Graph shows average ±s.e.m., n ≥60, * P <0.05 versus control (Student’s t -test). Full size image The current model of excretory canal development combines coalescence and fusion of vacuoles, activity of ion channels and aquaporins, cytoskeletal rearrangements and endocytic trafficking [8] , [9] , [10] . Endosomes, particularly through the slow recycling pathway, are critically important for facilitating plasma membrane building and subsequent maintenance. The trans -Golgi network (TGN) communicates with recycling endosomes (REs), providing secretory vesicles that contain proteins and lipids necessary for membrane building [11] . Endosomes sort the material and bud new vesicular carriers, which travel to and dock (with the aid of exocyst complexes) at the plasma membrane to unload their cargo. Surface material from the membrane is transported via endocytosis to endosomes, which sort and package the materials and membrane for return to the TGN. In this way, the endosomes and Golgi form a co-dependent relationship that sustains both the shape and function of the TGN and biogenesis of the TGN-derived vesicles, while promoting plasma membrane assembly and maintenance [11] . The small GTPase CDC-42 has been strongly implicated in regulating vesicle trafficking to and from Golgi [12] , [13] , [14] . Changes in the levels of signalling and structural proteins lead to defects in excretory canals. For example, loss-of-function mutations in the CDC-42 guanine nucleotide-exchange factor EXC-5 causes formation of large cysts in the apical membrane. In contrast, overexpression of EXC-5 causes canal truncations that arise through defects in the basolateral membrane [15] . Likewise, loss of the cytoskeletal linker Ezrin Radixin and Moesin family orthologue ERM-1 results in canal truncation and cyst formation, whereas overexpression causes severely widened lumen and cytoplasmic trailing at the distal tips [8] . Hence, maintaining the proper balance of small GTPase activity and cytoskeletal protein levels is critical for coordinating lumen formation and subsequent basolateral membrane addition during seamless tube extension. CCM is a neurovascular disease that can arise in an autosomal dominant manner (familial) or sporadically by unknown mechanisms [16] . Both familial and sporadic CCM are characterized by defects in brain capillaries that develop into enlarged ‘mulberry-like’ cysts (that is, clustered, fluid-filled, aberrations in the plasma membrane). Defective cell–cell junctions in these lesions cause blood to leak into the brain, leading to symptoms such as headaches, seizures and stroke in the most severe cases [16] . Three causative genes for familial CCM have been identified, which encode distinct scaffold proteins KRIT1 ( CCM1 ), malcavernin ( CCM2 ) and PDCD10 ( CCM3 ) [17] , [18] , [19] , [20] , [21] . Loss of the CCM1 gene, the most common genetic lesion in familial CCM, results in hyperactivation of RhoA and the Rho-activated kinase (ROCK), which culminates in stress fibre formation and compromised cell–cell junctions [22] . Although the three CCM proteins can form a ternary complex [23] , recent studies indicate that the majority of cellular CCM3 resides in the striatin interacting phosphatase and kinase complex (STRIPAK) and that CCM3 functions independently of CCM1 and CCM2 (refs 24 , 25 , 26 , 27 , 28 ). Critically, patients with mutations in the CCM3 gene have an earlier onset of disease, often during childhood, and more severe neurovascular defects [29] , supporting the idea that CCM3 may act by a mechanism that is distinct from CCM1 and CCM2. We show here that the C. elegans CCM3/PDCD10 orthologue CCM-3 and its binding partners, germinal centre kinase III (GCK-1) and striatin (CASH-1) promote extension of excretory canals during post-embryonic development. Furthermore, CCM-3 and GCK-1 localize to the apical canal membrane, and their ablation causes severe canal truncation and cyst formation. We find that CCM-3 functions in a cell-autonomous manner to promote CDC-42 signalling and RE integrity, independent of the CCM1/KRIT1 orthologue KRI-1. Using transmission electron microscopy (TEM) we show that ccm-3 loss-of-function mutants have defects in both basolateral and apical canal membranes. Apical defects, caused by dysregulated CV dynamics, result in formation of fluid-filled ectopic lumens (cysts) that resemble the ‘mulberry-like’ lesions of human CCM. These studies reveal a novel in vivo mechanism of action for CCM-3 as part of STRIPAK, which may help explain the more aggressive nature of this disease in patients harbouring mutations in the CCM3 gene. Loss of CCM-3 affects excretory canal morphology To investigate the biological function of CCM3 in a genetically tractable multicellular organism, we identified the C. elegans orthologue C14A4.11 (henceforth referred to as ccm-3 ), which encodes a protein of 215 amino acids that is 38% homologous to the mammalian protein [30] . To determine the expression pattern of CCM-3, we obtained a transgenic strain (BC13892) that contains a multicopy array expressing a transcriptional green fluorescent protein (GFP) reporter using 2,995 bp of the ccm-3 promoter [31] . Strong GFP signal was detected in the excretory canals, vulva and intestine ( Fig. 1c ). Using the same promoter we generated a single-copy integrant expressing a CCM-3::GFP fusion protein and observed localization along luminal membranes of the intestine, pharynx and germline that recapitulated the expression pattern of the transcriptional reporter in all tissues except the excretory canals ( Supplementary Fig. 1a–c ). We suspect that endogenous CCM-3 is maintained at low levels in the canal owing to its toxic effects when overexpressed (see below). Using a canal-specific promoter ( exc-9 ) we found that a CCM-3::GFP translational reporter showed localization to the apical membrane ( Fig. 1d ), confirmed by co-expression of the canal-specific basolateral marker CHC-1::mCherry ( Fig. 1e ). Extra-chromosomal arrays often overexpress proteins in C. elegans [32] . We observed that transgenic animals with markedly brighter signal (likely due to an overexpression of CCM-3::GFP) coincided with canals possessing distinctly widened lumens ( Fig. 1d —third panel). We also observed frequent (>50%) enrichment of CCM-3, displayed as bright spots and short trails at the tips of healthy extending canals ( Supplementary Fig. 1d ). To assess the biological function of ccm-3 , we examined the phenotype of a ccm-3 deletion allele ( tm2806 ). The tm2806 allele is a 442-base deletion that removes the second and third exons, and part of the forth exon, of the ccm-3 gene. This allele is predicted to generate a protein of 52 amino acids that is out of frame after amino-acid 25 and is likely a null allele since most of the N-terminal region required for interaction with its binding partner GCK-1 is removed [25] , [30] (see below). Homozygous ccm-3(tm2806) mutants are sterile and develop slower than wild-type (WT) animals. Given the importance of CCM genes in vascular development, we investigated a potential role for CCM-3 in excretory canals by introducing a canal-specific reporter (P vha-8 ::GFP) into ccm-3(tm2806) mutants. While ccm-3 heterozygotes (marked as ‘+/−’) did not have defective canals ( Fig. 1f ), homozygous mutants (marked as ‘ − /−’) had canal truncations to ~65% of their WT lengths ( Fig. 1g,l ). Truncations in ccm-3(− /−) worms were observed as early as the L3 larval stage of development, and the severity progresses into the adult stage, indicating an important role for CCM-3 in continuous post-embryonic excretory canal development. In addition, the existing canals exhibited multiple defects, including discontiguous (unconnected) lumen ( Fig. 1h , top panel), or otherwise ectopic lumen separate from the primary lumen, which were confirmed through Z-stack analysis. Also common was widening of the lumen, presence of cysts ( Fig. 1h , middle panel) and swollen cytoplasmic vesicles ( Fig. 1h , bottom panel) that perturb the basolateral membrane. At the distal tip, as well as long thin trails of cytoplasmic material ( Fig. 1i , top panel), lumenal cysts were also readily observed ( Fig. 1i , middle and bottom panels). These defects are present in ~95% of ccm-3(− /−) mutants, with cysts in over 40% ( Supplementary Table 1 ). Canal integrity worsens as the mutant animals age, taking the form of numerous fluid-filled bubble-like enlargements in the lumen ( Fig. 1i , middle panel) and enlarged vesicles in the cytoplasm that severely distort the basolateral membrane. Introducing WT ccm-3 under the control of its endogenous promoter rescued canal truncations and cysts in ccm-3(− /−) ( Fig. 1j ). Furthermore, ablation of ccm-3 by RNA interference (RNAi) completely recapitulated canal truncations seen in ccm-3(tm2806) homozygotes ( Fig. 1l ). To determine whether CCM-3 promotes canal extension by a cell-autonomous mechanism, we used the canal-specific translational reporter to express CCM-3 in ccm-3(− /−) worms. This rescued canal truncations and cysts ( Fig. 1k ), but not sterility, indicating that ccm-3 acts in a cell-autonomous manner to promote canal extension and integrity. We observed CCM-3::GFP overexpression in ~20% of these transgenic worms, which caused defects such as severe canal truncations, expanded lumens and strong cystic profiles ( Supplementary Fig. 1e ). Overexpression did not, however, change the apical localization of CCM-3 ( Supplementary Fig. 1f ). Similar defects have been reported by overexpression of canal structural proteins [8] , [10] . The C. elegans genome contains homologues for two human CCM genes ( kri-1 / CCM1 and ccm- 3/ CCM3 ). We previously identified a non-autonomous role for the CCM1 orthologue kri-1 in promoting germline apoptosis [33] . No canal defects were observed in kri-1 mutants ( Supplementary Fig. 2a ), supporting an emerging view that CCM3 has functions that are distinct from CCM1 and CCM2 (ref. 28 ). Using a KRI-1::GFP reporter ( Supplementary Fig. 2b ), previously shown to be expressed in the pharynx and intestine ( Supplementary Fig. 2c,d ) [33] , [34] , we confirmed that kri-1 is not detectably expressed in the excretory canals. Consistent with ccm-3 and kri-1 having distinct biological functions, we found that their co-ablation also results in synthetic lethality ( Supplementary Fig. 2e ). GCK-1 interacts with CCM-3 and promotes canal extension The C-terminal domains of each of the three GCKIII kinases (MST4, STK24 and STK25), the human orthologues of GCK-1, were previously shown to interact with the amino terminus of CCM3, and the critical residues required for contact are conserved in the worm proteins [30] . To determine whether worm CCM-3 and GCK-1 can also interact physically, we tagged these proteins with FLAG and GFP epitopes (respectively) and expressed them in HEK293T cells. Indeed, CCM-3 and GCK-1 physically interact, as shown by co-immunoprecipitation assays ( Fig. 2a ). Our canal-specific translational reporter for GCK-1 exhibited localization along the apical membrane, as well as the cytoplasm ( Fig. 2b ). Consistent with the biochemical data, we observed strong co-localization between GCK-1 and CCM-3 along the apical membrane of the canal ( Fig. 2c ). 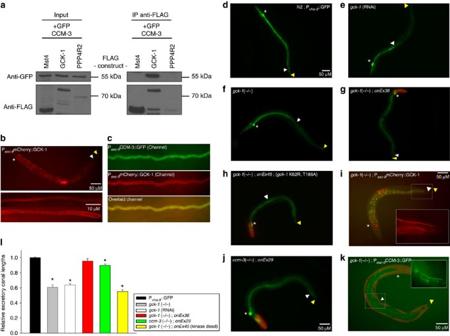Figure 2: CCM-3 promotes canal extension through GCK-1. (a) Co-immunoprecipitation of FLAG-tagged GCK-1 and GFP-tagged CCM-3 in HEK293T cells. Mst4 is the murine orthologue of GCK-1 that interacts with mammalian CCM3 ref.30, but notC. elegansCCM-3. PPP4R2 is a human phosphatase-associated protein that does not interact with human STRIPAK and is used here as a negative control. (b) A translational reporter for GCK-1 indicates strong presence along the apical membrane and in the cytoplasm. (c) GCK-1 co-localizes with CCM-3 in the canal. (d) Canals in wild-type background extend to full length of the body, compared with truncations after cultivating wild-type worms ongck-1(RNAi)(e) or ingck-1(−/−) (f), which have canal truncations to ~60% of control lengths (l). Expression of wild-type GCK-1 (g) but not a kinase dead mutant (h) from its endogenous promoter (transgenic animals indicated by the red signal of co-injection marker in the pharynx) rescued truncated canals ingck-1(−/−). Loss of GCK-1 was rescued by canal-specific GCK-1 overexpression (region marked by an inset box) (i), indicating cell autonomy. Overexpression of wild-type GCK-1 inccm-3(−/−) rescued canals back to wild-type lengths (j,l), indicating that CCM-3 promotes canal extension through catalytically active GCK-1. CCM-3 overexpression, however, could not rescue loss of GCK-1 (region marked by an inset box) (k). Asterisks denote location of the excretory cell (at the anterior/head of the worm). White and yellow arrowheads denote canal and total worm length, respectively. All canals are oriented from anterior (left) to posterior (right).b(top),d–k are at × 100 magnification;b(bottom),cand insets are at × 630 magnification. Graph shows average ±s.e.m.,n≥20, *P<0.05 from control (Student’st-test). Figure 2: CCM-3 promotes canal extension through GCK-1. ( a ) Co-immunoprecipitation of FLAG-tagged GCK-1 and GFP-tagged CCM-3 in HEK293T cells. Mst4 is the murine orthologue of GCK-1 that interacts with mammalian CCM3 ref. 30 , but not C. elegans CCM-3. PPP4R2 is a human phosphatase-associated protein that does not interact with human STRIPAK and is used here as a negative control. ( b ) A translational reporter for GCK-1 indicates strong presence along the apical membrane and in the cytoplasm. ( c ) GCK-1 co-localizes with CCM-3 in the canal. ( d ) Canals in wild-type background extend to full length of the body, compared with truncations after cultivating wild-type worms on gck-1(RNAi) ( e ) or in gck-1(− /−) ( f ), which have canal truncations to ~60% of control lengths ( l ). Expression of wild-type GCK-1 ( g ) but not a kinase dead mutant ( h ) from its endogenous promoter (transgenic animals indicated by the red signal of co-injection marker in the pharynx) rescued truncated canals in gck-1(− /−). Loss of GCK-1 was rescued by canal-specific GCK-1 overexpression (region marked by an inset box) ( i ), indicating cell autonomy. Overexpression of wild-type GCK-1 in ccm-3(− /−) rescued canals back to wild-type lengths ( j , l ), indicating that CCM-3 promotes canal extension through catalytically active GCK-1. CCM-3 overexpression, however, could not rescue loss of GCK-1 (region marked by an inset box) ( k ). Asterisks denote location of the excretory cell (at the anterior/head of the worm). White and yellow arrowheads denote canal and total worm length, respectively. All canals are oriented from anterior (left) to posterior (right). b (top), d –k are at × 100 magnification; b (bottom), c and insets are at × 630 magnification. Graph shows average ±s.e.m., n ≥20, * P <0.05 from control (Student’s t -test). Full size image Ablation of gck-1 by mutation or RNAi caused similar canal truncations and cyst formation as observed in ccm-3(− /−) ( Fig. 2e,f ). Canal truncations in gck-1(− /−) were rescued by a gck-1(+) transgenic array expressed from its endogenous promoter ( Fig. 2g,l ). To determine whether its kinase activity is required for tube extension, we generated a transgenic strain expressing a mutant GCK-1 containing amino-acid substitutions (K62R and T186A) that render it catalytically inactive [35] , [36] . This kinase dead mutant failed to rescue canal truncations when expressed in gck-1(− /−) worms ( Fig. 2h,l ), supporting a catalytic role for GCK-1 in promoting canal elongation. To assess autonomy, and determine whether gck-1 acts downstream of ccm-3 , we injected the canal-specific mCherry::GCK-1 translational reporter into gck-1(− /−) and ccm-3(− /−) worms, which restored canals to normal lengths in both genetic backgrounds ( Fig. 2i,j ). Conversely, expression of CCM-3 could not rescue canal defects of gck-1(− /−) mutants ( Fig. 2k ). These results indicate that the kinase activity of GCK-1 is necessary for canal elongation, and that it functions genetically downstream of CCM-3. CCM-3 affects CDC-42 activity and REs Mammalian CCM1 and CCM2 proteins negatively regulate the small guanine nucleotide-exchange factor RhoA to maintain vascular integrity [22] , [37] . Whether small GTPases are regulated by CCM3 is less clear [37] , [38] , [39] . In the C. elegans excretory system, ablation of the CDC-42-activating guanine-exchange factor EXC-5 causes severe canal truncations and cyst formation, possibly through defects in endocytic recycling [10] ( Fig. 3a ). Loss of rab-11 , a critical small GTP-binding protein that associates with REs and plays a key role in vesicle trafficking, causes canal truncations ( Fig. 3b , top panel), cyst formation and discontiguous lumen ( Fig. 3b , bottom panel) that resemble ccm-3(− /−) phenotypes. We therefore wished to address whether CCM-3 was implicated in the regulation of CDC-42. To do this, we monitored its localization using CDC-42::mCherry and its activation using GBDwsp-1::mCherry translational reporters [10] . In WT animals, these markers appear as punctate cytoplasmic bodies distributed along the length of canals ( Fig. 3c–g ; Supplementary Table 2 ). In ccm-3(− /−), we observed a striking reduction in CDC-42 and activated CDC-42 puncta ( Fig. 3c,d ). 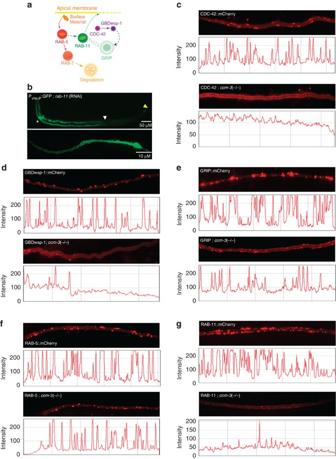Figure 3: CCM-3 promotes CDC-42 signalling and endocytic recycling. (a) Model of endocytic recycling in the excretory canal. Labels indicate vesicular compartments and signalling molecules studied with specific marker lines. Material is shuttled from the apical membrane into early endosomes (RAB-5). The path to degradation, via late endosomes (RAB-7), is marked with solid arrows. The path to material recycling linked to membrane growth through recycling endosomes (RAB-11), in contact with thetrans-Golgi network (GRIP), and mediated by CDC-42 signalling (GBDwsp-1 indicates active CDC-42), is marked with dashed arrows. (b) The importance of recycling is shown through loss ofrab-11, which causes canal truncation as well as significant lumenal defects and perturbations to the basolateral membrane (bottom panel). (c–f) Top panels show canal expression of the indicated mCherry-tagged proteins (forming punctuate bodies) in wild-type versus homozygousccm-3mutants (bottom panel). Below canal images are fluorescence intensity traces along the respective canals, where peaks indicate puncta of the tagged marker protein. Presence of CDC-42 and its activated form (c,d) are severely reduced in the absence ofccm-3. Golgi bodies (represented by the GRIP::mCherry marker) (e) are also diminished, indicating that CCM-3 is required for Golgi presence (or stability) along canals. While loss ofccm-3does not affect distribution and abundance of RAB-5 (early endosomes) (f), the lack of intact Golgi may also affect endocytic recycling, as indicated by diminished RAB-11::mCherry (g) puncta.b(top) is at × 100 magnification.b(bottom) andc–gshow posterior regions of the canal at × 630 magnification. All canals are oriented from anterior (left) to posterior (right). Figure 3: CCM-3 promotes CDC-42 signalling and endocytic recycling. ( a ) Model of endocytic recycling in the excretory canal. Labels indicate vesicular compartments and signalling molecules studied with specific marker lines. Material is shuttled from the apical membrane into early endosomes (RAB-5). The path to degradation, via late endosomes (RAB-7), is marked with solid arrows. The path to material recycling linked to membrane growth through recycling endosomes (RAB-11), in contact with the trans -Golgi network (GRIP), and mediated by CDC-42 signalling (GBDwsp-1 indicates active CDC-42), is marked with dashed arrows. ( b ) The importance of recycling is shown through loss of rab-11 , which causes canal truncation as well as significant lumenal defects and perturbations to the basolateral membrane (bottom panel). ( c – f ) Top panels show canal expression of the indicated mCherry-tagged proteins (forming punctuate bodies) in wild-type versus homozygous ccm-3 mutants (bottom panel). Below canal images are fluorescence intensity traces along the respective canals, where peaks indicate puncta of the tagged marker protein. Presence of CDC-42 and its activated form ( c , d ) are severely reduced in the absence of ccm-3 . Golgi bodies (represented by the GRIP::mCherry marker) ( e ) are also diminished, indicating that CCM-3 is required for Golgi presence (or stability) along canals. While loss of ccm-3 does not affect distribution and abundance of RAB-5 (early endosomes) ( f ), the lack of intact Golgi may also affect endocytic recycling, as indicated by diminished RAB-11::mCherry ( g ) puncta. b (top) is at × 100 magnification. b (bottom) and c – g show posterior regions of the canal at × 630 magnification. All canals are oriented from anterior (left) to posterior (right). Full size image Because mammalian CDC-42 is required for endocytic trafficking, a process that is known to be critical for canal development [10] , we asked whether CCM-3 affects early, late and/or RE markers. We introduced fluorescent markers of the Golgi (GRIP::mCherry), early endosome (RAB-5::mCherry) and RE (RAB-11::mCherry) into ccm-3(− /−) ( Fig. 3a,e–g ). Ablation of ccm-3 did not affect early or late endosomes (RAB-7::mCherry), but caused a severe dispersal of Golgi ( Fig. 3e,f ; Supplementary Fig. 3e ) and diminished RE reporter signals ( Fig. 3g ), which are normally distributed throughout the canal in WT animals [10] . The phenotypes in ccm-3(− /−) were phenocopied by RNAi ( Supplementary Fig. 3 ), suggesting that CCM-3 promotes a CDC-42-dependent endocytic recycling process. CCM-3 is required for membrane integrity Canal truncations and cyst formation that occur in later stages of larval development of ccm-3 mutants may indicate a breakdown of canal maintenance during its extension. To determine ultrastructural features of defective excretory canals in ccm-3 mutants, we viewed serial cross-sections of canals using TEM. There were striking structural changes at both the basolateral and apical membranes in canals of ccm-3(− /−) compared with WT animals ( Fig. 4a,b ). Whereas WT canals are generally round with organized apical and basolateral membranes, ccm-3(− /−) showed distinctive projections off the basolateral membrane and enlarged lumen ( Fig. 4b ). While both rough ER and Golgi bodies were readily observed within the cytoplasm of WT canals ( Fig. 4a ), they were rarely observed in ccm-3(− /−) canals although mitochondria were observed in both ( Fig. 4a,b ; Supplementary Table 3 ). Indeed, while there were significant reductions in Golgi/ER even in the anterior-most sections, mitochondria were seen more frequently in ccm-3 mutant worms ( Supplementary Table 3 ), although this is likely due to a static number of mitochondria dispersed throughout a much shorter tube. Distinctively, ccm-3(− /−) canals contain more than double the number of CVs compared with WT ( Fig. 4e ). The increased CV number was accompanied by an increase in lumen diameter that led to a doubling of lumen volume ( Fig. 4e ). Loss of ccm-3 appears to prevent normal CV incorporation into the lumen that drives canal development, similar to the dysregulation of cytoskeletal proteins (and organizers, such as ERM-1) [8] , [9] . Despite the shared phenotype of CV aggregation, loss of ccm-3 did not change ERM-1 localization, nor could overexpression of ERM-1 rescue ccm-3 mutant phenotypes ( Supplementary Fig. 4 ), which suggests that CCM-3 may act independently of ERM-1. 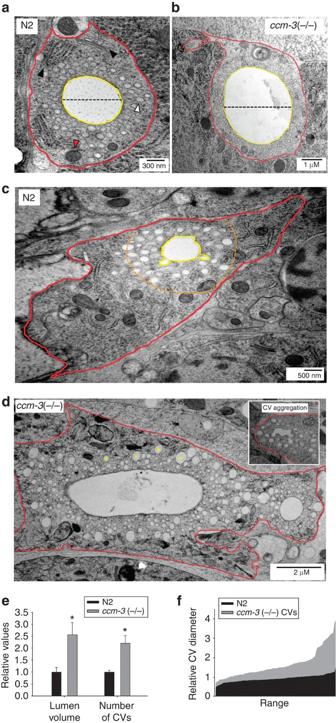Figure 4:ccm-3mutant canals have expanded lumen and increased canalicular vesicles. (a) Canals from wild-type worms display continuous and rounded basolateral membranes (marked in red) with similarly rounded apical/luminal (marked in yellow) membranes. In contrast, theccm-3mutant canal (b) shows a projection from the basolateral membrane, along with an expanded lumen (lumen diameters indicated with a dashed line). Arrowheads in the control canal (a) indicate Golgi and rough endoplasmic reticulum (solid black), mitochondria (red) and CVs (white); there are no visible Golgi/ER structures inccm-3mutant canals. (c) Developing canals often exhibit ‘bulbs’ of accumulated canal material (cytoplasm, organelles and so on) known as varicosities. Within these, the lumen size and number of CVs do not change. The dotted orange line indicates the approximate size of a standard N2 worm canal. (d) Heavily cystic canals (fromccm-3mutants) contain ectopic lumen (inset indicating nonspecific CV aggregation) and enlarged CVs (indicated by yellow asterisks). Quantification indicates that both lumen volume and number of CVs are doubled (e) (graph shows average ±s.e.m.,n=5, *P<0.05 (Student’st-test)) inccm-3mutant canals. CV size show great variability inccm-3mutant canals compared with wild-type controls (f) (n=100). All canal images were taken towards the anterior of the worm, within 100 μm of the excretory cell body at × 19,000 magnification (exceptd; × 6,500 magnification). Figure 4: ccm-3 mutant canals have expanded lumen and increased canalicular vesicles. ( a ) Canals from wild-type worms display continuous and rounded basolateral membranes (marked in red) with similarly rounded apical/luminal (marked in yellow) membranes. In contrast, the ccm-3 mutant canal ( b ) shows a projection from the basolateral membrane, along with an expanded lumen (lumen diameters indicated with a dashed line). Arrowheads in the control canal ( a ) indicate Golgi and rough endoplasmic reticulum (solid black), mitochondria (red) and CVs (white); there are no visible Golgi/ER structures in ccm-3 mutant canals. ( c ) Developing canals often exhibit ‘bulbs’ of accumulated canal material (cytoplasm, organelles and so on) known as varicosities. Within these, the lumen size and number of CVs do not change. The dotted orange line indicates the approximate size of a standard N2 worm canal. ( d ) Heavily cystic canals (from ccm-3 mutants) contain ectopic lumen (inset indicating nonspecific CV aggregation) and enlarged CVs (indicated by yellow asterisks). Quantification indicates that both lumen volume and number of CVs are doubled ( e ) (graph shows average ±s.e.m., n =5, * P <0.05 (Student’s t -test)) in ccm-3 mutant canals. CV size show great variability in ccm-3 mutant canals compared with wild-type controls ( f ) ( n =100). All canal images were taken towards the anterior of the worm, within 100 μm of the excretory cell body at × 19,000 magnification (except d ; × 6,500 magnification). Full size image During development, the canal contains beaded projections at intervals along its length called varicosities ( Fig. 4c ). These varicosities contain an abundance of cytoplasmic material and organelles that are thought to provide membrane and proteins for canal extension. Although there is an accumulation of cytoplasmic material in varicosities of WT worms, there is no change in CV abundance or lumen diameter. Hence, part of the cystic phenotype (ectopic lumen formation and cytoplasmic vesicle swelling) of ccm-3 mutants is likely due to improper CV aggregation, which may be exacerbated by the addition of vesicles derived from fragmented Golgi ( Fig. 4d ). Many of these vesicles are expanded in size and can be up to four times the width of the uniform-sized WT CVs ( Fig. 4f ). Further, TEM images reveal hyper-aggregated CVs that apparently generate ectopic lumen ( Fig. 4d , inset). This may result from the rate of vesicle fusion events exceeding that of endocytic recycling, as suggested by Kolotuev et al. [9] To assess the progression of canal defects along its length, we sampled multiple short regions, at 50-μm intervals, with serial sections ( Supplementary Fig. 5a ). Canals in WT worms were uniform in shape, size and organelle content along their lengths ( Supplementary Fig. 5b ). In contrast, ccm-3(− /−) canals exhibited substantial basolateral membrane protrusions, as well as an expanded and progressively more damaged lumen towards the distal (posterior) tips ( Supplementary Fig. 5c ). In addition, rough ER and Golgi bodies were only observed in the anterior-most section of ccm-3(− /−) canals, and absent from the posterior sections ( Supplementary Fig. 5c , top panel). This is consistent with our observations using the GRIP::mCherry Golgi marker ( Fig. 3e ). Therefore, canal defects in ccm-3 mutants exhibit a progressively more severe phenotype towards their distal tips. GCK-1/STRIPAK promotes canal elongation In mammals the core STRIPAK complex is assembled via direct interactions between the striatin scaffold, protein phosphatase PP2A and CCM3, which recruits GCKIII class kinases [25] . Several other molecules of poorly characterized function also assemble on this well-defined core phosphatase and kinase module [25] , [40] , [41] . The cash-1 , farl-11 , C30A5.3 and C49H3.6 genes encode worm orthologues of striatin, STRIP1/2, MOB3 and CTTNBP2/NL, respectively ( Fig. 5a ; Supplementary Table 4 ) [40] . With the exception of MOB3 and CTTNBP2/NL, ablation of every component of the predicted C. elegans STRIPAK complex caused truncations in canals, similar to ccm-3(− /−) ( Fig. 5b–f ; Supplementary Table 4 ). We also asked whether ablating GCK-1 or other STRIPAK components affected endocytic recycling in a similar manner as CCM-3. In the absence of gck-1 ( Fig. 5g–j , middle panels) or cash-1 ( Fig. 5g–j , bottom panels) there was a drastic reduction in CDC-42, activated CDC-42, as well as reduced presence of Golgi and REs ( Supplementary Table 2 ). 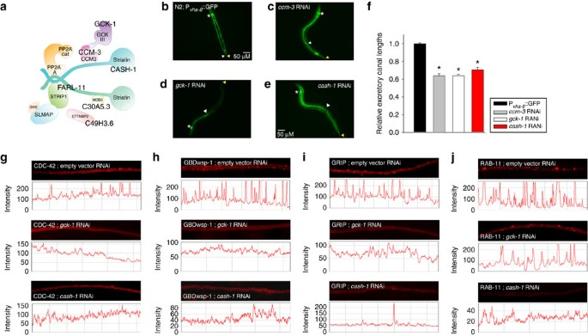Figure 5: STRIPAK promotes canal extension and endocytic recycling. (a) The STRIPAK complex is composed of multiple interacting proteins that are conserved inC. elegans(indicated in bold). Compared with N2 controls (b), ablation of core STRIPAK genesccm-3(c),gck-1(d), theC. elegansstriatin orthologuecash-1(e) andfarl-11/STRIP1/2 caused similar canal truncations (f,Supplementary Table 4). (g–j) RNAi to empty vector (top),gck-1(middle) andcash-1(bottom), respectively. Ablation of STRIPAK components by RNAi atteunated CDC-42 signalling (g,h), as indicated by reduced puncta. The presence of Golgi (i) and recycling endosomes (j) were similarly reduced by ablation ofgck-1andcash-1. Asterisks denote location of the excretory cell (at the anterior/head of the worm), white and yellow arrowheads denote canal and total worm length, respectively.b–eare at × 100 magnification;g–jare at × 630 magnification. All canals sections are taken from the same region, oriented from anterior (left) to posterior (right). Truncations range from ~30 to 40% from controls (b). Graph shows average ±s.e.m.,n≥20, *P<0.05 from control (Student’st-test). Figure 5: STRIPAK promotes canal extension and endocytic recycling. ( a ) The STRIPAK complex is composed of multiple interacting proteins that are conserved in C. elegans (indicated in bold). Compared with N2 controls ( b ), ablation of core STRIPAK genes ccm-3 ( c ), gck-1 ( d ), the C. elegans striatin orthologue cash-1 ( e ) and farl-11 /STRIP1/2 caused similar canal truncations ( f , Supplementary Table 4 ). ( g – j ) RNAi to empty vector (top), gck-1 (middle) and cash-1 (bottom), respectively. Ablation of STRIPAK components by RNAi atteunated CDC-42 signalling ( g , h ), as indicated by reduced puncta. The presence of Golgi ( i ) and recycling endosomes ( j ) were similarly reduced by ablation of gck-1 and cash-1 . Asterisks denote location of the excretory cell (at the anterior/head of the worm), white and yellow arrowheads denote canal and total worm length, respectively. b – e are at × 100 magnification; g – j are at × 630 magnification. All canals sections are taken from the same region, oriented from anterior (left) to posterior (right). Truncations range from ~30 to 40% from controls ( b ). Graph shows average ±s.e.m., n ≥20, * P <0.05 from control (Student’s t -test). Full size image Given the reported similarity in loss of RAB-11 with a loss of the exocyst complex, which tethers vesicles arriving from the Golgi to the plasma membrane [42] , [43] , [44] , we wondered whether the exocyst was also required for canal integrity. We introduced the vha-8 ::GFP canal marker in a strain carrying the exoc-8(ok2523) deletion allele and observed moderate canal truncations ( Supplementary Fig. 6a,d ), while loss of ccm-3 in conjunction with exoc-8 did not exacerbate these defects beyond truncations observed in ccm-3 single mutants ( Supplementary Fig. 6b,d ). Despite a relatively moderate truncation effect, exoc-8 mutants exhibited extremely strong cystic profiles ( Supplementary Fig. 6c ), in agreement with a recent report [45] . Along with apical cysts at the canal tip ( Supplementary Fig. 6c , right panels), discontiguous lumen, enlarged cytoplasmic vesicles and perturbed basolateral membranes were frequently observed. It is possible, given the effect of CCM-3 on recycling components that EXOC-8 and CCM-3 cooperate to promote trafficking. CDC-42 regulates canal length and Golgi/RE integrity Following our observations of reduced CDC-42 presence with ablation of CCM-3 and other STRIPAK components, we asked whether CDC-42 was required for canal extension. Ablation of cdc-42 by mutation or RNAi caused truncations and canal cyst formation similar to loss of ccm-3 ( Fig. 6a ). Furthermore, ablation of cdc-42 reduced Golgi and RE markers to a similar extent as loss of ccm-3 ( Fig. 6d–g , middle panels; Supplementary Table 2 ). To test the specificity of CDC-42 in promoting canal extension, we inhibited other small GTPases, rho-1 (RhoA) and chw-1 (RhoU/RhoV) by RNAi and observed no effects on WT canals ( Supplementary Fig. 7a,b ). Given the role of CCM3 (in its complex with CCM1 and CCM2) in repressing RhoA activity [4] , [22] , we asked whether rho-1 ablation could restore canal length or RE puncta in ccm-3(− /−). Loss of rho-1 had no discernable effect on canal length nor on RAB-11 puncta in ccm-3(− /−) worms ( Supplementary Fig. 7c ), positioning CDC-42 as the main Rho GTPase effector of the putative C. elegans CCM3–STRIPAK signalling pathway. 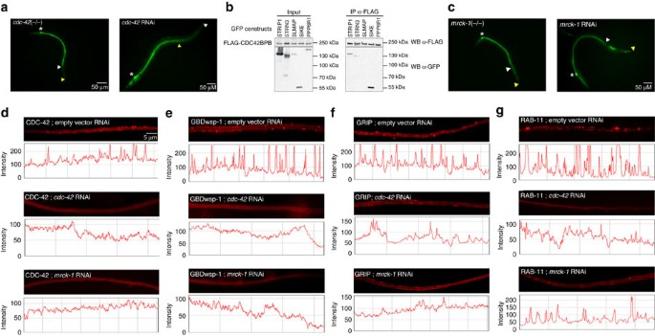Figure 6: CDC-42 and MRCK-1 affect canal growth and endocytic recycling. (a) Mutation (left) and RNAi (right) to the Rho GTPasecdc-42cause similar canal truncations and cysts. (b) CDC42BPB (aka MRCKβ) co-immunoprecipitated (i) with multiple STRIPAK complex components in mammalian cells. (c) TheC. elegansMRCK orthologuemrck-1(left—mutant; right—RNA) also caused canal truncations and cysts when ablated. (d–g) RNAi to control empty vector (top),cdc-42(middle) andmrck-1(bottom), respectively. CDC-42 signalling (d,e), Golgi (f) and recycling endosomes (g) puncta are dispersed by RNAi tocdc-42andmrck-1. Asterisks denote location of the excretory cell (at the anterior/head of the worm). White and yellow arrowheads denote canal and total worm length, respectively.aandcare at × 100 magnification;d–gare at × 630 magnification. Canal sections are taken at the same region of the posterior canal, oriented from anterior (left) to posterior (right). Figure 6: CDC-42 and MRCK-1 affect canal growth and endocytic recycling. ( a ) Mutation (left) and RNAi (right) to the Rho GTPase cdc-42 cause similar canal truncations and cysts. ( b ) CDC42BPB (aka MRCKβ) co-immunoprecipitated ( i ) with multiple STRIPAK complex components in mammalian cells. ( c ) The C. elegans MRCK orthologue mrck-1 (left—mutant; right—RNA) also caused canal truncations and cysts when ablated. ( d – g ) RNAi to control empty vector (top), cdc-42 (middle) and mrck-1 (bottom), respectively. CDC-42 signalling ( d , e ), Golgi ( f ) and recycling endosomes ( g ) puncta are dispersed by RNAi to cdc-42 and mrck-1 . Asterisks denote location of the excretory cell (at the anterior/head of the worm). White and yellow arrowheads denote canal and total worm length, respectively. a and c are at × 100 magnification; d – g are at × 630 magnification. Canal sections are taken at the same region of the posterior canal, oriented from anterior (left) to posterior (right). Full size image Activation of RhoA upon loss of CCM proteins leads to the formation of actin stress fibres [22] . Given the roles of actin in vesicular transport and TGN dynamics, we next asked whether increasing the pool of available actin could rescue loss of ccm-3 . Introducing an extra-chromosomal array that overexpresses ACT-5::GFP into the ccm-3(− /−) worms caused a fourfold increase in full rescue (canal length >90%, relative body length) compared with ccm-3(− /−) ( Supplementary Fig. 8 ). Interestingly, the number of RAB-11 puncta in rescued canals increased slightly ( Supplementary Table 2 ), suggesting that CCM-3 may promote endocytic recycling, in part through effects on actin organization. MRCK-1 is required for canal extension Proteomic analysis of STRIPAK interacting proteins in human cells identified the CDC-42-binding protein (CDC42BPB), also known as the myotonic dystrophy-related CDC-42-binding kinase (MRCK), as another putative CCM3 interactor (J.D.R.K., M.G. and A.-C.G., unpublished data). Physical interaction between CDC-42-binding proteins and several STRIPAK components was recapitulated by immunoprecipitation coupled to immunoblotting ( Fig. 6b ). Given the role of MRCK in the regulation of CDC-42 signalling [46] , [47] , which has also been reported in C. elegans [48] , we asked whether the C. elegans CDC42BPB/MRCK orthologue MRCK-1 was required for canal development. Ablation of mrck-1 by mutation or RNAi caused canal truncations and cyst formation that resembled the effect of ccm-3 , gck-1 , STRIPAK or cdc-42 ablation ( Fig. 6c ). Similar to ablation of CCM-3, STRIPAK and CDC-42, we observed a strong dispersal of the Golgi reporter and a reduction in both REs and CDC-42/GBDwsp-1 ( Fig. 6d–g , bottom panels; Supplementary Table 2 ). These results suggest that CCM-3 and STRIPAK promote seamless tube extension, in part through CDC-42/MRCK-1, revealing a new role for MRCK in this process. Elucidating how integrity of biological tubes is maintained has important implications in development, and our understanding of CCM disease, where brain capillaries develop malformations that can severely disable affected patients [16] . Our results are consistent with an emerging view that CCM3 also functions independently of CCM1 and CCM2. While the three vertebrate CCM proteins can form a ternary complex, with CCM2 acting as a hub to bind both CCM1 and CCM3 (refs 23 , 49 , 50 ), the apparent absence of a CCM2 gene in C. elegans may explain the distinct functions of KRI-1 and CCM-3. Importantly, we show that ccm-3 is critical for tube growth, and furthermore, that it functions by a cell-autonomous mechanism, although it is interesting to note that CCM3 can function both autonomously and non-autonomously in vertebrates [26] . The localization of CCM-3 to the apical membrane, and subsequent apical membrane defects (that is, enlarged lumen and significant accumulation of CVs in the cytoplasm), as well as frequent enrichment at the growing distal tip, reveal a conserved role for this protein in vascular tube extension and maintenance. In mammalian cells CCM3 and its binding partners, the germinal centre kinases (MST4/STK24/STK25), are tightly associated with the STRIPAK complex and are required for Golgi polarization [25] , [40] . Studies in murine and fly models have suggested different roles for CCM3 and GCKIII in biological tube development: promoting lumen formation in mice, and localizing junction and polarity proteins at the interface of multicellular and unicellular tubes in flies [38] , [51] . Growth of the terminal seamless tubes of Drosophila trachea are dependent on the regulation of small GTPases and vesicle trafficking, in which CCM3 and GCKIII have been implicated [51] , [52] . Here, we show that the C. elegans CCM3 and GCKIII orthologues ( ccm-3 and gck-1 ), in cooperation with STRIPAK, control seamless tube growth through CDC-42/MRCK-1-dependent regulation of endocytic recycling ( Fig. 7a ). 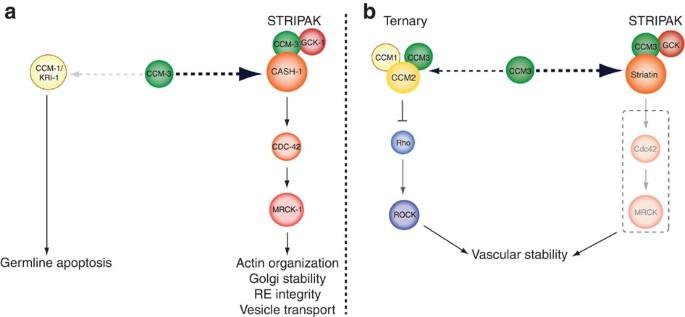Figure 7: Model. CCM-3/STRIPAK modulates CDC-42 signalling (ostensibly through MRCK-1) to correctly promote Golgi stability, RE integrity and vesicle transport. These roles are likely reliant on actin organization, and ultimately result in successful tube extension/maintenance. TheC. elegansCCM-3 (a) acts independently of KRI-1 (in the absence of a worm CCM2 orthologue), which has no apparent role in tube development, in contrast to the vertebrate model (b). This may indicate a conserved role of CCM3 fundamental to biological tube development. Figure 7: Model. CCM-3/STRIPAK modulates CDC-42 signalling (ostensibly through MRCK-1) to correctly promote Golgi stability, RE integrity and vesicle transport. These roles are likely reliant on actin organization, and ultimately result in successful tube extension/maintenance. The C. elegans CCM-3 ( a ) acts independently of KRI-1 (in the absence of a worm CCM2 orthologue), which has no apparent role in tube development, in contrast to the vertebrate model ( b ). This may indicate a conserved role of CCM3 fundamental to biological tube development. Full size image Although ablation of mammalian CCM1, -2 or -3 leads to upregulation of RhoA and ROCK [22] , [37] , [39] , [53] , our data suggest that CCM-3 and STRIPAK preferentially modulate CDC-42 signalling, posing the question of whether multiple CCM3 complexes collaborate to maintain vascular stability in vertebrates. Along with recent evidence indicating that CCM3 is predominantly associated with the STRIPAK complex [40] , the exceptional clinical aggressiveness caused by loss of CCM3 could be due to synergistic defects that arise from disruption of multiple complexes. To this point, a pathological form of CCM3 found in patients, which lacks 18 amino acids in the N-terminal region, can still form a ternary complex with CCM1–CCM2 but does not bind the GCKIII kinase [53] . Since CCM3 binds both STRIPAK [25] and CCM2 (ref. 54 ) through its C-terminal focal adhesion kinase-targeting domain, it is possible that the two independent CCM3 complexes co-exist. Therefore, CCM3 may function in two independent pathways that regulate distinct signalling cascades through RhoA and Cdc42 to promote vascular tube development and plasma membrane stability. What we observed in C. elegans may represent a primitive role for CCM-3 in vasculature development that has expanded in mammals ( Fig. 7 ). Consistent with a role for STRIPAK in regulating GTPase signalling, we found the mammalian STRIPAK complex also interacts with the CDC-42-binding kinase MRCK. Ablation of cdc-42 or mrck-1 in C. elegans causes canal truncations similar to ablation of ccm-3 or gck-1 . Furthermore, punctate CDC-42 is dispersed, supressing the presence of active CDC-42 at the distal tip when ccm-3 , gck-1 , mrck-1 and cash-1 are ablated. Since we did not observe any significant canal defects after rho-1 silencing, we favour a model in which CCM-3 and STRIPAK preferentially act through CDC-42, at least in C. elegans . While the mammalian CCM1–CCM2 and CCM1–CCM2–CCM3 complexes have been shown to affect Rho signalling and actin polymerization, mammalian STRIPAK proteins interact with Golgi, cytoskeletal components and proteins involved in vesicular trafficking [41] . Crucially, both complexes likely target the same process via separate signalling cascades, namely actin regulation. Given the well-established role of CDC-42 in regulating actin, and the roles of actin in Golgi shape/stability, vesicle formation, secretion and transport [13] , [55] , we propose that CCM-3 modulates the actin cytoskeleton via CDC-42/MRCK-1 ( Fig. 7a ). The partial rescue of ccm-3 mutant phenotypes by overexpression of actin supports this hypothesis, especially if loss of ccm-3 could divert available actin pools into stress fibres. Recent work showing differential effects on the actin cytoskeleton by ROCK and MRCK at endothelial cell junctions highlights the necessity to balance suppression of Rho/ROCK and activation of CDC-42/MRCK [56] . With excess Rho/ROCK activity, actin becomes tied up in stress fibres [22] , whereas CDC-42/MRCK promotes circumferential actin bundles critical for junction formation [56] . This may explain the functional split between CCM1˙CCM2˙CCM3 ternary and CCM3–STRIPAK complexes in vertebrates, if the modulation of CDC-42 by CCM-3 is conserved ( Fig. 7 ). The apparent downregulation of endocytic recycling (reduction in RAB-11) that we observe with loss of ccm-3 may arise through defects in Golgi integrity via the actin cytoskeleton. Indeed, Golgi-associated CDC-42 promotes vesicle formation by modulating actin polymerization [57] , and is the only Rho GTPase known to regulate Golgi function [58] . Hence, where both ER and Golgi are significantly diminished in ccm-3(− /−) canals, defects in cytoskeleton-mediated transport of these organelles is not likely responsible since mitochondria are still present. Rather, we suspect a specific defect in Golgi (and possibly ER) stability. Fragmentation of the ER and Golgi manifests as an increased presence of vesicles [59] , [60] , making them hard to discern from other vesicles, such as CVs. Perhaps some of the larger vesicles we detected in the EM sections of ccm-3(− /−) canals represent the fragmented products of ER and Golgi. Fragmentation of the Golgi may also reduce the RE integrity, which could contribute to loss of apical membrane integrity. Rab11 regulates apical REs [61] , [62] , and its depletion in mammalian cells caused improperly localized accumulation of REs (often to the basolateral membrane), preventing functional apical recycling. This concurs with the apical phenotypes we see with loss of rab-11 , and supports the idea that CCM-3 promotes endocytic recycling. Loss of Rab11 can also affect the exocyst complex by binding Sec15, which helps mediate communication with endocytic vesicles [44] . Both CCM-3 and the exocyst localize to the apical membrane, and the exocyst has been shown to promote lumenogenesis through vesicle fusion [45] , [63] . However, we are uncertain as to whether CCM-3 might act directly on the exocyst, through RAB-11, or even another protein, to affect vesicle fusion. In neutrophils, for example, CCM3 promotes exocytosis through the small GTPase Rab27 (ref. 64 ). In summation, it is becoming clear that CCM3 regulates multiple trafficking events, many of which are likely to be cell-type specific. Ultrastructural analysis revealed a number of defects in the ccm-3 mutant canal such as aggregation of CVs, ectopic lumen, abnormal lumen expansion and basolateral membrane perturbations. The basolateral perturbations, while potentially a result of defective recycling/exocytosis, are more likely due to vesicle accumulation and radial lumen expansion. The variation in the individual CV diameter in the heavily cystic canals may reflect their nature as channels, through which hydrostatic pressure can be generated [8] , [9] . Expanding CVs (and possibly vesicles derived from fragmented Golgi/ER) may mechanically push the cytoplasmic contents against the membrane, causing the observed basolateral projections. The CV aggregation and enlarged lumen phenotype is particularly reminiscent of ERM-1 overexpression [8] . While there is evidence that CCM3-associated GCKIII and MRCK can phosphorylate ERM [65] , [66] , we remain cautious of suggesting a direct interaction here, since loss of ccm-3 did not appear to affect levels or localization of ERM-1, nor could functional ERM-1 restore full-length canals. Hence, where ERM-1 is integral to early development of the canal [8] , our observations are more consistent with those of Song et al. [51] , showing that CCM3 defects do not prevent lumen formation per se , but rather lead to dilations through improper addition of membrane. This study brings together concepts from several model systems pointing to a novel mechanism by which CCM-3, in association with STRIPAK, influences small GTPase signalling (CDC-42 and RAB-11) to maintain Golgi stability and endocytic recycling. The disease state of CCM3 mutation is widely recognized as the most severe, and as such, we propose that CCM3 functions concurrently within two complexes to balance GTPase signalling and maintain plasma membrane stability. Our observations in the C. elegans excretory canal, along with mammalian conservation in CCM-3 and STRIPAK interactions, may provide insights into intrinsic mechanisms by which cavernous malformations develop in CCM patients, and help identify drug targets for alleviating or reversing CCMs. C. elegans strains and maintenance Worms were cultivated on lawns of Escherichia coli (strain OP50) grown on nematode growth medium plates at 20 °C (unless otherwise stated) [67] . The following strains were provided by the Caenorhabditis Genetics Centre: BC13892, CF2282, RB1928, WH556 and JS345. The unbalanced ccm-3(tm2806)/+ strain was originally obtained from the Japanese National Bioresource Project. WT refers to the C. elegans variety Bristol, strain N2. See Supplementary Table 5 for the strain list. All excretory canal marker strains were a kind gift from Dr Matthew Buechner. The ERM-1::GFP and ACT-5::GFP strains were a kind gift from Dr Verena Göbel. DNA constructs and microinjection Extra-chromosomal-rescuing arrays were generated by microinjection of a construct containing 3.2 kb of the ccm-3 promoter and the WT ccm-3 gene (including introns) cloned into the pCFJ151 vector, then co-injected with pCFJ90 (P myo-2 ::mCherry) and pGH8 (P rab-3 ::mCherry) into ccm-3(tm2806) / mIn1 (strain WD188) worms. The gck-1 -rescuing array was generated by isolating the WT gck-1 gene and 1.8 kb of promoter from fosmid WRM0622bf08 and co-injected with pCFJ90 (P myo-2 ::mCherry) into gck-1(km15) / nT1 worms (strain WD195). Canal-specific rescue of ccm-3 (strain WD382) and gck-1 (strain WD420) was achieved by replacing the mCherry gene in pBK162 (a kind gift from Dr Matthew Buechner) with ccm-3 complementary DNA (cDNA). The pBK162 vector contains the exc-9 promoter to drive canal-specific expression. This rescuing plasmid was co-injected with pBK162 and pCFJ90 into ccm-3(tm2806) / mIn1 worms (strain WD188). The CCM-3::GFP translational reporter was constructed by cloning the P exc-9 promoter, ccm-3 and gfp cDNAs into a pUC19 backbone. This construct was injected into N2, WD119 and JS345 and BK219 strains to generate strains listed in Supplementary Table 5 . The GCK-1::mCherry translational reporter was constructed by cloning gck-1 cDNA into the pBK162 vector (containing both P exc-9 and mCherry). This construct was injected into JS345, WD119 and co-injected with the CCM-3 translational reporter into N2 worms (see Supplementary Table 5 ). Microinjection was performed using a FemtoJet (Eppendorf) microinjections system attached to an inverted Leica DMI3000B microscope. RNA interference RNAi was performed by feeding bacteria expressing double-stranded RNA (RNAi), from the Source Bioscience LifeSciences feeding library, to worms at the L1 stage. RNAI bacteria, was streaked onto LB media plates (with ampicillin and tetracycline), and incubated for 18 h at 37 °C. Individual colonies were selected with a sterile p200 tip, and were transferred to tubes containing liquid LB+ampicillin+tetracycline. These were grown for 24 h (at 37 °C) in an orbital shaker, prior to induction with isopropyl-b- D -thiogalactoside (0.1 M) for 4 h (37 °C, orbital shaker). RNAi was plated on RNAi media plates (containing isopropyl-b- D -thiogalactoside and carbenicillin) and left to grow at room temperature overnight. Worms were staged at L1 through hypochlorite bleaching. Overgrown plates (containing many eggs) were treated with hypochlorite bleach for 5 min at room temperature, before having the bleach transferred to Eppendorf tubes. The tubes were centrifuged at 2,000 r.p.m. for 1 min and were followed by two more bleach washes/centrifugation steps and three washes/centrifugation with M9 buffer. Eppendorf tubes, containing eggs in M9 buffer, were left for 24 h in a rotary mixer (at 20 °C), and L1s were plated the following day. In the case of essential genes (such as rab-11 ), it was necessary to plate the worms on RNAi at the L3 stage. Differential interference contrast (DIC) microscopy L4 and young adult-staged worms were slide mounted in a 5-μl aliquot of tetramisole anaesthetic (20 mM), on a flat pad of agar (4%). Nematodes were viewed with a Leica DMRA2 compound microscope equipped with epifluorescence and Nomarski optics. The images are marked for magnification individually. Images were captured with a Hamamatsu C472-95 digital camera using Openlab software (PerkinElmer Inc.). Images reflect a single plane. Typically only a single ‘arm’ of the canal can be seen, with the other (in a lower plane) obscured by the intestine. The canals imaged at × 100 and × 630 magnification were always selected on this basis of relative clarity. Canal lengths were measured from the pharynx to the tip of the canal and were calculated relative to body length, as measured from the terminal pharynx bulb to the anus. High-pressure freeze fixation and TEM L4 and young adult-staged worms were fixed with high-pressure freezing, followed by freeze substitution, in a procedure modified from Stigloher et al. [68] A total of 10–12 worms in OP50 bacteria were transferred into the cavity of the freezing chamber (specimen carriers type A (100 μm) and B (0 μm); Bal-Tec AG, acquired by Leica Microsystems) and processed by an EM HPM100 (Leica Microsystems); freezing speed >20,000 K s −1 , pressure >2,000 bar. The resultant frozen pellets were liberated from their carriers, directly into liquid nitrogen, to an EM AFS2 freeze substitution system (Leica Microsystems). Samples were fixed with 0.1% tannic acid and 0.5% glutaraldehyde in acetone (−90 °C for 96 h), and further washed four times for 1 h with acetone at −90 °C. The pellets were post-fixed with 2% osmium tetroxide in acetone (−90 °C for 28 h). The temperature was subsequently raised to −20 °C for 14 h, incubated for 16 h (still at −20 °C) and then raised again to 4 °C over 4 h. Pellets were washed with acetone (at 4 °C) four times at 30-min intervals. The temperature was increased to 20 °C over a period of 1 h and finally samples were embedded in a series of freshly prepared Araldite solutions. Here, concentrations increased from 50% Araldite in acetone (3 h at room temperature) to 90% Araldite in acetone (overnight at 4 °C), to pure Araldite at room temperature (two times). Araldite-treated samples were allowed to polymerize for 48 h at 60 °C. A total of 10–12 serial sections (90 nm per section) were taken at three sequential 50-μm intervals for both control (N2) and ccm-3(tm2806) homozygotes. Images of the excretory canal were obtained on FEI Tecnai 20 equipped with an AMT16000 digital camera. Statistical analyses Statistical significance of canal lengths were expressed as a percentage, and normalized to a value of 1 based on WT canals. All values in charts are mean±s.e.m. from three or more experimental data sets. P values were determined using a two-tailed Student’s t -test, assuming equal variance. Significance levels ( P value) and sample size ( N ) are marked in each corresponding figure legend. Puncta/fluorescent measures for endocytic/CDC-42 marker strains were conducted with Image J software using a Red, Green, Blue (RGB) profile plot on a stretch of canal (~100 μm in length) at or near the posterior distal tip. Each image shows a single plane, of one canal, with the maximal amount of puncta present. Relative intensity of the Red Fluorescent Protein (RFP or mCherry) was assessed, with puncta presence marked with peaks and non-punctate areas with troughs. Canal lumen volume, CV diameter and CV number measurements were conducted using ImageJ software (NIH); ccm-3 mutant data were normalized against N2 data to show relativity. Immunoprecipitation and immunoblotting The mouse pcDNA3-FLAG-Mst4 (BC005708), human pcDNA3-FLAG-PPP4R2 (NM_174907) and human pcDNA5-GFP-SLMAP (BC115701) constructs used were described previously [40] , [69] . C. elegans CCM3 (NM_063889) and human PPP6R1 (BC094753) were PCR amplified from cDNA with EcoRI and NotI added at the 5′ and 3′ ends, respectively. Following digestion with EcoRI and NotI, the inserts were introduced into pcDNA5/FRT/TO-eGFP. C. elegans gck-1 (NM_072908) was cloned similarly, except that it was inserted into pcDNA5-FLAG. Human CDC42BPB (NM_006035) in pENTR223 was obtained from the Dana-Farber/Harvard Cancer Center DNA Resource Core and recombined into pDest-pcDNA5-Flag using LR clonase. Human SIKE (BC005934), mouse Strip1 (BC023952) and human STRN3 (BC126221) were originally cloned in pcDNA3-FLAG [40] . Inserts for these genes were subsequently PCR amplified with attL1 and attL2 recombination sites added to the 5′ and 3′ ends, respectively. The PCR products were inserted into pDONR223 (Invitrogen) using BP clonase and then recombined into pcDNA5/FRT/TO-eGFP using LR clonase. All inserts were sequence verified. Immunoprecipitation and western blotting were performed as follows: low passage HEK293T cells were co-transfected using jetPRIME transfection reagent (Polyplus Cat# CA89129-924) as per the manufacturer’s protocol. Cells were lysed with 50 mM Hepes-KOH pH 8.0, 100 mM KCl, 2 mM EDTA, 0.1% NP40, 10% glycerol, 1 mM phenylmethylsulphonyl fluoride, 1 mM dithiothreitol and Sigma protease inhibitor cocktail (Cat# P8340) and subjected to passive lysis followed by one freeze–thaw cycle. Lysates were incubated with FLAG M2-agarose beads for 1.5 h, washed three times with lysis buffer and directly eluted by boiling in Laemmli buffer. Precipitated proteins were separated via SDS–polyacrylamide gel electrophoresis, transferred to nitrocellulose and detected with antibodies directed against the FLAG or GFP epitopes. These can be seen in Supplementary Fig. 9 . How to cite this article: Lant, B. et al. CCM-3/STRIPAK promotes seamless tube extension through endocytic recycling. Nat. Commun. 6:6449 doi: 10.1038/ncomms7449 (2015).